The ASIC3/P2X3 cognate receptor is a pain-relevant and ligand-gated cationic channel Two subclasses of acid-sensing ion channels (ASIC3) and of ATP-sensitive P2X receptors (P2X3Rs) show a partially overlapping expression in sensory neurons. Here we report that both recombinant and native receptors interact with each other in multiple ways. Current measurements with the patch-clamp technique prove that ASIC3 stimulation strongly inhibits the P2X3R current partly by a Ca 2+ -dependent mechanism. The proton-binding site is critical for this effect and the two receptor channels appear to switch their ionic permeabilities during activation. Co-immunoprecipation proves the close association of the two protein structures. BN-PAGE and SDS-PAGE analysis is also best reconciled with the view that ASIC3 and P2X3Rs form a multiprotein structure. Finally, in vivo measurements in rats reveal the summation of pH and purinergically induced pain. In conclusion, the receptor subunits do not appear to form a heteromeric channel, but tightly associate with each other to form a protein complex, mediating unidirectional inhibition. Acid-sensing ion channels (ASICs) belong to the epithelial sodium channel/degenerin (ENaC/DEG) family; they are gated by protons and exhibit a cationic permeability with marked preference for Na + over K + [1] , [2] . P2X receptors (Rs) are gated by adenosine triphosphate (ATP) and allow the passage of mono- and divalent cations with a roughly identical permeability for Na + and K + [3] , [4] . In spite of their different amino acid sequences, the two receptor types adopt a similar molecular structure (composition of three subunits; each subunit consists of two transmembrane segments, intracellular N and C termini, and a large extracellular loop; cavities and vestibules with deep negative electrostatic potentials in their extracellular domains; similar ion conductive pathways) [5] , [6] . In rodents, at least six ASIC subunits (ASIC1a, ASIC1b, ASIC2a, ASIC2b, ASIC3, ASIC4) encoded by four different genes have been described. They are able to associate into homomeric and heteromeric channels. The ASIC currents are activated transiently upon extracellular acidification; their activation threshold, pH sensitivity and current kinetics depend on the subunit composition. P2XRs are built up of 7 mammalian subunits (P2X1–7) encoded by the same number of genes; they also associate into homomeric or heteromeric receptor channels. The individual receptors differ in their pharmacological sensitivities towards agonists and antagonists as well as in their biophysical properties (single channel conductance, inward rectification, rapid or slow desensitization). ASICs are widely expressed throughout the pain pathways, both in the peripheral and central nervous systems [7] , [8] . Of these channels, ASIC1 and ASIC3 are the most sensitive to protons, being activated already by very small acidification. ASIC3 is present at dorsal root ganglion (DRG) neurons projecting to the spinal cord dorsal horn. This channel is supposed to mediate various pain qualities associated with a decrease of pH in the cellular interstitium of cutaneous or muscle tissue during inflammation, ischemia and cancer metastasis. The homomeric P2X3 and the heteromeric P2X2/3Rs both participate in the sensation of painful stimuli and are also located at DRG neurons [9] , [10] , [11] . They are involved in acute, inflammatory, neuropathic, visceral and cancer pain, which uniformly lead to an increased release of ATP into the extracellular space. P2XRs have been described to negatively interact with members of the Cys-loop receptor family such as nicotinic, GABA A/C and 5-HT 3A receptors [12] , [13] , [14] , [15] , [16] . This receptor crosstalk involves physical interaction between two ion channel proteins located in close proximity during simultaneous agonist application [17] , [18] . The proposed models commonly entail a general mechanism of state-dependent propagation of allosteric states in large multiprotein complexes. Through this ‘conformational spread’, the gating movements of one receptor are communicated to the other one and result in its closure. In view of the high structural similarity of ASIC3 and P2X3 receptor channels, and their co-localization in DRG neurons, we asked ourselves whether ASIC3/P2X3 subunits form a trimeric channel or whether the two receptors associate to a multiprotein complex. After identifying an inhibitory crosstalk between the two receptor types operating predominantly at low ATP concentrations, we coined the term ‘cognate receptor’. This term describes an extremely tight association of ASIC3 and P2X3Rs which results in unilateral depression of the P2X3R currents and the switch of their ionic conductance during activation by the respective agonists. Activation of recombinant ASIC and P2X3Rs in CHO cells In a first series of experiments, we decided to study the functional properties of co-expressed recombinant rat (r)ASIC3 and rP2X3Rs. The recombinant subunits were transiently transfected into Chinese hamster ovary (CHO) cells rather than HEK293 cells, because the latter cell type possesses endogenous ASICs [19] , inevitably interfering with our current measurements. This cell line is not listed as misidentified in the database of the International Cell Line Authentication Committee. Whole-cell membrane currents were determined in CHO-rASIC3 cells by means of the patch-clamp technique at a holding potential of −65 mV. The fast local change in pH by superfusing an external medium which had the same ionic composition but a different proton concentration than the control one induced a rapidly desensitizing inward current (Fig. 1a , upper panel). Then, we generated pH–response relationships by plotting the log proton concentration against the amplitude of the current response (pH 7.0–5.5, i.e. 0.1–3.16 µM H + ; Fig. 1b ). Similarly, we applied increasing concentrations of the P2X1,3R selective agonist α,β-methylene ATP (α,β-meATP; 0.3–300 μM) onto CHO-rP2X3 cells to construct a concentration–response curve (Fig. 1a , lower panel, Fig. 1c ). It is noteworthy that the I max value of the proton-induced current was considerably higher than that caused by α,β-meATP application (Fig. 1b, c and Suppl. Tables 1 , 2 ). Further, the ASIC3 curve was steeper than the P2X3R curve, and protons were more potent than α,β-meATP. The different Hill numbers ( n H ) suggest that protons occupied more agonist binding sites than α,β-meATP did (Suppl. Tables 1 , 2 ). Fig. 1 Concentration–response curves for agonists at various ASICs and P2X3Rs expressed in CHO cells. a – c Whole-cell patch-clamp recordings of proton and α,β-meATP-induced currents. Both types of agonists were applied at the indicated increasing concentrations for 2 s onto CHO cells transfected with rASIC3 ( a , upper panel) or rP2X3 ( a , lower panel). The intervals between individual applications were kept at 2 min (protons) or 5 min (α,β-meATP) in order to avoid the decrease of the subsequent current amplitudes by desensitization. Drug application procedures in this and all subsequent panels of this figure were identical. CHO cells expressing rASIC3 ( b ) or rP2X3 ( c ) were treated with amiloride (AMI; 10 µM) or A-31749 (10 µM) while constructing concentration–response curves. In this and all subsequent panels of this figure, means ± S.E.M. of the indicated number of experiments are shown. Broken lines represent curves obtained in response to agonist application to CHO cells containing ASIC3 or P2X3Rs only, in the absence of any additional drug. d – f CHO cells were transfected with rASIC3 and rP2X3 cDNA in a 1:1 ratio. Whole-cell patch-clamp recordings of proton and α,β-meATP-induced currents. Cells were treated with amiloride (10 µM) or A-31749 (10 µM) while constructing pH- or concentration–response curves. g – i CHO cells were transfected with hASIC3 alone or together with hP2X3 cDNA in a 1:1 ratio. Whole-cell patch-clamp recordings of proton and α,β-meATP-induced currents. Cells were treated with A-31749 (10 µM) while constructing pH- or concentration–response curves. j – l CHO cells were transfected with rASIC1a or rASIC2a alone or together with rP2X3 cDNA in a 1:1 ratio. Whole-cell patch-clamp recordings of proton-induced currents through rASIC1a ( j , upper panel, k ) or rASIC2a ( j , lower panel, l )-containing receptors. The holding potential was −65 mV in all experiments. * P < 0.05; statistically significant difference of the I mean values from the respective curves designated by broken lines at the highest agonist concentrations (one-way ANOVA followed by the Holm–Sidak test, or Student’s t -test, as appropriate). The scale labels for the vertical bars were 10 nA ( a , upper panel), 2 nA ( a , lower panel), 2 nA ( d ), 500 pA ( g ), 2 nA ( j , upper panel) and 10 nA ( j , lower panel). The scale labels for the horizontal bars were 20 s ( a , d , g , j ) Full size image Then, we designed experiments with the highly selective P2X3R antagonist A-317491 (10 μM) [20] and found that it did not alter the effect of protons, but depressed the effect of α,β-meATP (Fig. 1b, c ). By contrast, amiloride, an antagonist of the ENaC/DEG family of ion channels [21] , equally depressed the I max of the concentration–response curves for both protons and α,β-meATP (Fig. 1b, c , Suppl. Tables 1 , 2 ). This finding may indicate that both ASIC3 and P2X3Rs possess identical binding sites for amiloride, suggesting structural relationship. We co-transfected CHO cells with rASIC3 and rP2X3 in a 1:1 relationship in order to find out whether protons and α,β-meATP interact with each other in the presence of both receptors. It was a striking observation that the concentration–response curves of both protons and α,β-meATP were largely inhibited in the CHO-rASIC3/rP2X3R, in comparison with the CHO-rASIC3 and CHO-rP2X3R cells (Fig. 1d–f ; Suppl. Tables 1 , 2 ). A-317491 (10 μM) and amiloride (10 µM) acted in the doubly transfected cells in a similar manner as in their singly transfected counterparts. We found a marked difference between human and rat ASIC3 in the different ranges of pH values at which they are activated (Fig. 1g–i ; Suppl. 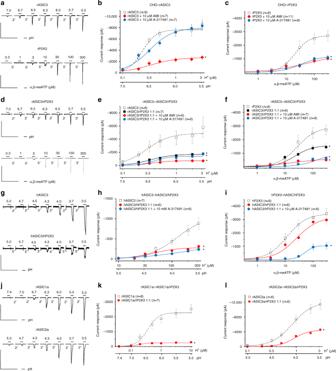Fig. 1 Concentration–response curves for agonists at various ASICs and P2X3Rs expressed in CHO cells.a–cWhole-cell patch-clamp recordings of proton and α,β-meATP-induced currents. Both types of agonists were applied at the indicated increasing concentrations for 2 s onto CHO cells transfected with rASIC3 (a, upper panel) or rP2X3 (a, lower panel). The intervals between individual applications were kept at 2 min (protons) or 5 min (α,β-meATP) in order to avoid the decrease of the subsequent current amplitudes by desensitization. Drug application procedures in this and all subsequent panels of this figure were identical. CHO cells expressing rASIC3 (b) or rP2X3 (c) were treated with amiloride (AMI; 10 µM) or A-31749 (10 µM) while constructing concentration–response curves. In this and all subsequent panels of this figure, means ± S.E.M. of the indicated number of experiments are shown. Broken lines represent curves obtained in response to agonist application to CHO cells containing ASIC3 or P2X3Rs only, in the absence of any additional drug.d–fCHO cells were transfected with rASIC3 and rP2X3 cDNA in a 1:1 ratio. Whole-cell patch-clamp recordings of proton and α,β-meATP-induced currents. Cells were treated with amiloride (10 µM) or A-31749 (10 µM) while constructing pH- or concentration–response curves.g–iCHO cells were transfected with hASIC3 alone or together with hP2X3 cDNA in a 1:1 ratio. Whole-cell patch-clamp recordings of proton and α,β-meATP-induced currents. Cells were treated with A-31749 (10 µM) while constructing pH- or concentration–response curves.j–lCHO cells were transfected with rASIC1a or rASIC2a alone or together with rP2X3 cDNA in a 1:1 ratio. Whole-cell patch-clamp recordings of proton-induced currents through rASIC1a (j, upper panel,k) or rASIC2a (j, lower panel,l)-containing receptors. The holding potential was −65 mV in all experiments. *P< 0.05; statistically significant difference of theImeanvalues from the respective curves designated by broken lines at the highest agonist concentrations (one-way ANOVA followed by the Holm–Sidak test, or Student’st-test, as appropriate). The scale labels for the vertical bars were 10 nA (a, upper panel), 2 nA (a, lower panel), 2 nA (d), 500 pA (g), 2 nA (j, upper panel) and 10 nA (j, lower panel). The scale labels for the horizontal bars were 20 s (a,d,g,j) Table 1 ). Thus, the pH 50 value of hASIC3 was 3.9, whereas that of rASIC3 was 6.6. These results are in contradiction to results published earlier which showed that the pH 50 values of human and rat ASIC3 were identical [22] . However, the difference in the range of pH values needed for activation may be due to the fact that we used in the present study the isoform ‘b’ of the hASIC3 instead of the isoform ‘a’ that was described by De Weille et al. [22] . The two isoforms differ from each other in the C-terminal 30 amino acids. Nevertheless, in the present experiments protons had a larger I max on hASIC3 expressed alone than when co-expressed with hP2X3, and the selective P2X3R antagonist A-317491 (10 µM) did not alter the effect of protons (Fig. 1h ) in accordance with similar experiments carried out with the rat orthologs of the two receptor channels (Fig. 1b ). Further, the transfection of hP2X3 and hASIC3/hP2X3 into CHO cells yielded receptor channels with similar sensitivities to α,β-meATP; in this case A-317491 (10 µM) markedly depressed the effect of α,β-meATP on the co-transfected channel (Fig. 1i ). These results again largely agreed with data generated on the rat orthologs of the human ASIC3/P2X3R (Fig. 1c ). Subsequently, we turned our attention to rASIC1a and rASIC2a. rASIC1a was activated in the same range of pH values as rASIC3 (Fig. 1k ), whereas rASIC2a exhibited a pH threshold which was higher than that of rASIC3 (Fig. 1l ). Nonetheless, co-transfection of these ASICs with P2X3 produced strong downward displacements of the pH–response curves with a corresponding depression of their I mean values (Fig. 1j–l ). Interaction between the two recombinant receptors It is interesting to note that in the CHO-rASIC3/rP2X3 cell population, the pre-application of protons (pH 6.7 or 6.5 instead of the normal 7.4) induced a rapidly desensitizing inward current, and 10 s later a pH-dependent depression of the α,β-meATP (10 µM) current response (Fig. 2a , lower panel, Fig. 2b ). A similar, although less pronounced, inhibition was observed at pH 6.5, when the concentration of α,β-meATP was increased to 100 µM (Fig. 2c ). In control measurements, cells were transfected with rP2X3 only. In these experiments, acidification of the pH value from 7.4 to 6.5 failed to alter the effect of α,β-meATP (10 µM; Fig. 2d , lower panel, Fig. 2f ). When the pH was kept throughout at pH 7.4, there was no change in the α,β-meATP-induced current responses over time either in the CHO-rASIC3/rP2X3 or in the CHO-rP2X3 cell population (Fig. 2a, d , upper panels, Fig. 2f ). The inhibitory interaction between protons and α,β-meATP was strictly unilateral; although the effect of pre-applied α,β-meATP (10, 30 µM) also rapidly desensitized in the continuous presence of this agonist, there was no consequent depression of the current responses to repeatedly applied protons (pH 6.5; Fig. 2e, g ). Fig. 2 Interaction between rASIC3 and rP2X3Rs after their transfection into CHO cells. CHO cells were transfected with rASIC3 and rP2X3Rs in a 1:1 ratio or transfected only with rP2X3R as indicated. Whole-cell patch-clamp recordings at a holding potential of −65 mV. a – c Interaction between rASIC3 and rP2X3Rs on their sequential activation by agonists. Current responses were elicited by α,β-meATP (10 or 100 µM) for 2 s with 5 min intervals before, during and after a shift in pH from 7.4 to 6.7 or 6.5. The reproducibility of the responses to α,β-meATP after changing to a solution with the same pH of 7.4 is also shown. d , f No effect of protons on rP2X3Rs. Current responses were elicited by α,β-meATP (10 µM) for 2 s with 5 min intervals before, during and after a shift in pH from 7.4 to 6.5. e , g No effect of α,β-meATP (10 and 30 µM) on the proton-induced inward current on the sequential activation of rP2X3 and rASIC3Rs. Stable responses to pH 6.5 in the absence of α,β-meATP is also shown. Percentage changes of α,β-meATP (10 and 100 µM)-induced current responses were calculated with respect to the second current before the pH shift to 6.7 or 6.5 ( b , c , f ). Percentage changes of proton (pH 6.5)-induced current responses were calculated with respect to the second current amplitude before the application of α,β-meATP (0, 10 and 30 µM) ( g ). Means ± S.E.M. of the indicated number of experiments. * P < 0.05; statistically significant difference between the current amplitudes before and after the long-lasting shift in pH or the long-lasting presence of α,β-meATP (one-way ANOVA followed by the Bonferroni test). The scale labels for the vertical bars were 500 pA ( a ) and 2 nA ( d , e ). The scale labels for the horizontal bars were 50 s ( a , d , e ) Full size image The inhibitory interaction between rASIC3 and rP2X3Rs has also held true for the human orthologs. In fact, pre-superfusion with a low pH external medium (pH 3.5) depressed the effect of α,β-meATP (10 µM) in perfect agreement with experiments on rASIC3/rP2X3Rs (compare Fig. 2a–c with Fig. 3a, b ). In the following experiments, we investigated whether rP2X3Rs also modulate currents through other rASICs (e.g., rASIC1a or rASIC2a) than rASIC3. However, of the two ASIC channels investigated, only the activation of rASIC1a depressed the effect of α,β-meATP (10 µM; Fig. 3c, d ). Fig. 3 Interaction between various ASICs and P2X3Rs after their transfection into CHO cells. CHO cells were transfected with various ASICs and P2X3Rs in a 1:1 ratio or transfected only with rP2X3R or rASIC3, as indicated. Whole-cell patch-clamp recordings at a holding potential of −65 mV. a , b Interaction between hASIC3 and hP2X3Rs on their simultaneous activation. Interaction between rASIC1a ( c ) or rASIC2a ( d ) with rP2X3Rs on their simultaneous activation. The drug application and evaluation protocols were like those used in Fig. 2a–g . Means ± S.E.M. of the indicated number of experiments. * P < 0.05; statistically significant difference between the current amplitudes before and after the shift in pH. § P < 0.05; statistically significant difference between the pH-induced inhibition of the current amplitudes at pH 4.0 and 3.5 (one-way ANOVA followed by the Bonferroni test in both cases). e Current responses were elicited in CHO-rASIC3/rP2X3R cells by α,β-meATP (10 µM) before, during and after the application of GMQ. f Means ± S.E.M. percentage changes of the α,β-meATP-induced current responses were calculated with respect to the second current amplitude before GMQ application. g Inhibition of current responses to α,β-meATP in CHO-rP2X3R cells. h Means ± S.E.M. percentage inhibition in the indicated number of experiments as shown in ( g ). i No change of the GMQ (1 mM)-induced current in the presence of α,β-meATP (10 µM) in CHO-rASIC3 cells. j Means ± S.E.M. percentage change in the indicated number of experiments as shown in ( i ). * P < 0.05; statistically significant difference from the α,β-meATP-induced current amplitudes before GMQ application (one-way ANOVA followed by the Bonferroni or Mann–Whitney test, as appropriate). The scale labels for the vertical bars were 2 nA ( a , g , i ) and 1 nA ( e ). The scale labels for the horizontal bars were 50 s ( a , e , g , i ) Full size image The depression of the α,β-meATP (10 µM) effect by the activation of rASIC3 was strictly limited to the occupation of the proton-binding site(s). When the non-proton-site activator 2-guanidine-4-methylquinazoline (GMQ; 1 mM) [23] was superfused for 10 s, a long-lasting non-desensitizing opening of the channel occurred (Fig. 3e, f ). α,β-meATP (10 µM) applied in the continuous presence of GMQ caused a rapid and reversible blockade of the GMQ-induced steady-state current (Fig. 3e, f ). Thus, GMQ strongly inhibited the α,β-meATP current (or increased its rate of desensitization), although not via an ASIC3/P2X3R interaction, because a decrease of α,β-meATP (10 µM)-induced currents also occurred in cells transfected with rP2X3 only (Fig. 3g, h ). Additional experiments showed that in cells transfected with rASIC3 rather than with rP2X3, α,β-meATP (10 µM) failed to interact with the GMQ (1 mM)-induced current (Fig. 3i, j ). Hence, α,β-meATP acted via P2X3Rs when interfering with the GMQ current. Finally, it can be concluded that in double-transfected cells the proton-site activation is a prerequisite for ASIC3/P2X3R interaction. Then, we changed the extracellular Ca 2+ concentration ([Ca 2+ ] o ) from the normal 2 mM to 0 or 4 mM to investigate the accompanying modulation of the rASIC3 and rP2X3R currents. The intracellular Ca 2+ concentration ([Ca 2+ ] i ) was also modified either by decreasing the buffering capacity of EGTA in the pipette solution (only 1.1 mM instead of the normal 11 mM) or by increasing the speed and capacity of buffering (instead of 11 mM EGTA, 5 mM BAPTA). Whereas modifications of [Ca 2+ ] o or [Ca 2+ ] i into either direction depressed the proton-induced currents (Fig. 4a, b ), these manipulations did not appreciably alter the α,β-meATP-induced currents (Fig. 4c, d ) in cells transfected either with rASIC3 or with rP2X3. When the interaction between protons and α,β-meATP was studied with the standard protocol in CHO-rASIC3/rP2X3 cells, both a no and a high Ca 2+ -containing external medium decreased/abolished the inhibitory effect of protons at pH 6.7 and 6.5 on the α,β-meATP-induced currents observed at normal [Ca 2+ ] o (Fig. 4e ). Similarly, both low and high Ca 2+ -containing pipette solutions interfered with the effect of protons on the α,β-meATP currents in comparison with the situation at a normal [Ca 2+ ] i (Fig. 4f ). Thus, changes in the extra- and intracellular concentrations of Ca 2+ modified the unilateral interaction of rASIC3 with rP2X3Rs, suggesting a dependence on Ca 2+ . Fig. 4 Changes in the Ca 2+ concentration modify rASIC3 and rP2X3R currents in CHO cells. Whole-cell patch-clamp recordings at a holding potential of −65 mV. a , b Concentration–response curves for protons in CHO cells transfected with rASIC3. a Inhibitory effect of an increase or decrease of the Ca 2+ concentration in the external medium ([Ca 2+ ] o ). b Inhibitory effect of an increase or decrease of the free Ca 2+ concentration in the patch pipette solution ([Ca 2+ ] i ). c , d Concentration-response curves for α,β-meATP in CHO cells transfected with rP2X3. c No effect of changes in [Ca 2+ ] o . d No effect of changes in [Ca 2+ ] i . Means ± S.E.M. of the indicated number of experiments. * P < 0.05; statistically significant difference of the I mean values at the highest agonist concentration (one-way ANOVA followed by the Holm–Sidak test). e , f CHO cells transfected with both rASIC3 and rP2X3 in a 1:1 ratio. Modulation of the unilateral interaction between rASIC3 and rP2X3Rs, by changes in [Ca 2+ ] o ( e ) and [Ca 2+ ] i ( f ); the experimental protocol is identical to that shown in Fig. 2a . * P < 0.05; statistically significant difference from the current amplitudes measured in normal extra- and intracellular Ca 2+ . § P < 0.05; statistically significant difference between currents at pH 6.7 or 6.5 at different Ca 2+ concentrations (one-way ANOVA followed by the Bonferroni test). Concentration–response relationships for protons ( g ) and α,β-meATP ( h ) in CHO-rASIC3/rP2X3R cells, in the absence and presence of J-8 (30 µM). Means ± S.E.M. of the indicated number of experiments. * P < 0.05; statistically significant difference between the I mean values at the highest agonist concentration (Student’s t -test). i Potentiation of the α,β-meATP (30 µM) current by co-application with a J-8 (30 µM)-containing, low pH (6.5) external medium, but inhibition in the absence of J-8 by acidification; representative tracings. j Percentage changes of α,β-meATP-induced current responses were calculated with respect to the second current amplitude before the pH shift. Means ± S.E.M. of the indicated number of experiments. * P < 0.05; statistically significant difference between the current amplitudes before and after the pH shift from 7.4 to 6.5 in the presence of J-8. § P < 0.05; statistically significant difference between current amplitudes at pH 6.5 in the presence or absence of J-8 (Mann–Whitney test). The scale labels for the vertical and horizontal bars in ( i ) were 1 nA and 50 s, respectively Full size image Under the assumption that Ca 2+ acts via Ca 2+ -sensitive intracellular messengers, we used the calmodulin antagonist J-8. J-8 (30 µM) decreased the I max of the concentration–response curves both for protons and α,β-meATP in cells co-transfected with rASIC3/rP2X3 (Fig. 4g, h , Suppl. Tables 1 , 2 ). Furthermore, J-8 turned the inhibitory effect of acidification to pH 6.5 on the α,β-meATP (10 µM) current into potentiation (Fig. 4i, j ) indicating at least partial receptor interaction by a Ca 2+ /calmodulin-dependent kinase. The next question to be answered was whether in our expression system rASIC3 and rP2X3 constitute a heterotrimeric receptor, e.g., consisting of 1 rASIC3 and 2 rP2X3 subunits, or whether two independent receptors interact with each other. It was expected that the reversal potential ( E rev ) of the supposed ASIC3/P2X3 heteromeric receptor channel, activated by either agonist, would be located somewhere between the reversal potentials of the two homomeric channels. To clarify this issue, we first determined the E rev for protons (pH 6.5) in CHO-rASIC3 cells and found it to be 50.1 ± 3.3 mV ( n = 10; Fig. 5a , left panel). The subsequent determination of the E rev for α,β-meATP (10 µM) in CHO-rP2X3R cells yielded −3.9 ± 3.4 mV ( n = 6; Fig. 5a , middle panel). Then, we applied consecutively the two agonists (protons followed by α,β-meATP) onto CHO cells co-transfected with both receptor channels (1:1 relationship of their complementary DNAs (cDNAs)) and determined their E rev (Fig. 5a , right panel). However, this procedure resulted in current responses with E rev values of −10.8 ± 4.4 mV ( n = 6) and 43.2 ± 2.9 mV ( n = 6), respectively. In order to substantiate this unexpected finding, we measured the E rev of the two agonists in separate populations of CHO-ASIC3/P2X3R cells and were able to confirm the switch of the reversal potential (protons, −5.8 ± 4.4 mV, n = 7; α,β-meATP, 47.1 ± 4.2 mV, n = 6) (Fig. 5c , left and right panels, respectively). Further, blockade of the ASIC3 channel activity by its selective antagonist APETx2 (0.1 µM) in doubly transfected cells shifted the E rev of α,β-meATP to a value of −14.9 ± 3.1 mV ( n = 6; Fig. 5d ), somewhat more negative than that measured in cells transfected with P2X3Rs only. The E rev values of the membrane currents were calculated from the current–voltage curves shown in Fig. 5b, d . Fig. 5 Switch of reversal potentials between co-expressed rASIC3 and rP2X3Rs in CHO cells. Whole-cell patch-clamp recordings at a holding potential of −65 mV. a Current traces induced by protons (pH 6.5) and α,β-meATP (10 µM) applied individually onto CHO-rASIC3 (left panel) and CHO-rP2X3R cells (middle panel) or successively onto CHO-rASIC3/P2X3 cells (right panel). Agonist application was at holding potentials which increased stepwise from −60 to + 90 mV in 30 mV increments. Current–voltage relationships were constructed from recordings similar to those shown in ( a ) in order to determine the reversal potentials ( E rev ) ( b ). Means ± S.E.M. of the indicated number of experiments. c Measurement of E rev of protons (left panel) and of α,β-meATP (right panel) by a similar protocol as shown in ( a ) on separate populations of CHO-rASIC3/rP2X3R cells. Under these conditions, the E rev values of these two agonists were interchanged. Current–voltage relationships constructed from recordings similar to those shown in ( c ) in order to determine the E rev ( d ). Means ± S.E.M. of the indicated number of experiments. Blockade of ASIC3 channel activity by the selective antagonist APETx2 (0.1 µM) shifted the E rev of α,β-meATP back near to its original value of around 0 mV. e In CHO-rASIC3/rP2X3R cells, ramps of 200 mV duration (−90 to  +90 mV) were delivered at a holding potential of −65 mV to determine the E rev of ASIC3 after a drop of the normal pH from 7.4 to 6.5. Then, a high concentration of α,β-meATP (100 µM) was applied in order to change the distribution of extra- and intracellular ions. Eventually, the E rev was re-determined after washing out α,β-meATP. Original tracing; large capacitive artifacts at the beginning and end of the ramp-induced currents were retouched. f Current–voltage curves were constructed from the indicated number of experiments similar to that shown in ( e ). The scale labels for the vertical bars were 2 nA ( a , left panel), 1 nA ( a , middle and right panels), 1 nA ( c ) and 500 pA ( e ). The scale labels for the horizontal bars were 1 s ( a , c ) and 2 s ( e ) Full size image These experiments indicated that α,β-meATP and protons have in singly transfected CHO cells two clearly discernible reversal potentials, one at about 0 mV (characteristic for non-selective cationic currents) and the other one somewhat below +65 mV (characteristic for Na + currents under our experimental conditions). In cells transfected with both ASIC3 and P2X3, the application of protons and α,β-meATP did not cause an identical ionic permeability but appeared to result in a switch of the reversal potential values between the two receptor channels. Although it could be hypothesized that even at pH 7.4 a small number of sustained leaky ASIC3 channels may alter the distribution of cations between the intra- and extracellular space which thereby causes a spurious change in the reversal potential of P2X3Rs, this did not seem to be the case (see below). To measure safely E rev , it is assumed that the concentrations of ions on either side of the membrane do not change, and the shift of E rev signals a change in membrane permeability to one or both ions (here ASIC3 exhibits a marked preference for Na + over Cs + which replaced K + in the pipette solution). An alternative hypothesis is that a shift in reversal potential reflects changes in ion concentrations (for P2X2Rs see ref. [24] ). In order to exclude this possibility, we used a protocol similar to that of Li et al. [24] and delivered to CHO-rASIC3/rP2X3R cells ramps of 200 mV duration from −90 to +90 mV from a holding potential of −65 mV to determine the E rev of ASIC3 after a drop of the normal pH from 7.4 to 6.5 (Fig. 5e, f ). The respective current–voltage curve yielded E rev at about 0 mV (0.3 ± 6.6 mV; n = 9) instead of the expected ASIC3-typical value of about +65 mV. The subsequent application of a high concentration of α,β-meATP (100 µM), which should cause a redistribution of ions between the intra- and extracellular sides of the membrane, shifted E rev of the ASIC3 current to the left (−36.6 ± 5.7 mV; n = 9; P < 0.05). Thus, a consecutive application of protons and α,β-meATP might not be a reliable method to determine in the same experiment the respective reversal potentials, especially at concentrations of α,β-meATP (100 µM instead of 10 µM) higher than used by us. Therefore, separate populations of ASIC3/P2X3R-CHO cells were utilized to determine individually the E rev of protons and α,β-meATP (see above; Fig. 5c, d ). In conclusion, when the expression system contained both receptors, the function of the selectivity filters of the two receptor channels appeared to be modified by their close proximity, resulting in a switch of the respective ionic conductances. Up to this point we clarified that rASIC3 can interact with the co-expressed rP2X3Rs in that the two receptor channels have a lower ionic permeability than each channel alone (Fig. 1d–f ). We speculated that, in addition, the activation of rASIC3 may decrease the ability of α,β-meATP to occupy the binding pouch of rP2X3Rs. Alternatively, rASIC3 may interfere with the gating movement of rP2X3Rs after agonist binding in order to depress the inhibitory interaction between the two receptors. In an attempt to discriminate between these possibilities, the following experiments were designed. We used dominant negative binding site mutants of rP2X3 in which particular lysine moieties were replaced by alanine (K63A, K299A) [25] , [26] . Supplementary Fig. 1a confirms that the replacement of either lysine moiety abolished the α,β-meATP current in CHO-rP2X3R-mut cells. However, these mutants failed to alter the depression of the α,β-meATP-induced maximal current in the CHO-ASIC3/P2X3R-mut cells in comparison with their wild-type counterpart (Suppl. Fig. 1b ). Moreover, variations in the ASIC3/P2X3R-mut ratio (1:2, 1:1, 1:4) emphasized the significance of P2X3R to determine the extent of the inhibitory effect imposed upon ASIC3 (Suppl. Fig. 1c,d ). Nonetheless, these experiments unequivocally documented that the ATP-binding site has no significance for the attenuation of the I max of the proton-induced current in CHO-ASIC3/P2X3R vs. CHO-ASIC3 cells. Further, we have reported previously that spontaneous tightening of the binding jaw of P2X3Rs by inter-subunit cross-linking of cysteine residues substituted at positions not directly involved in agonist binding inhibited the agonist-evoked currents due to a constraint of the conformational flexibility of the agonist binding jaw [27] . Figure 6a, b shows that when the K201C/V274C double mutant of the rP2X3R was transfected into CHO cells, the reducing agent dithiothreitol (DTT; 1 mM) increased the effect of α,β-meATP (10 µM), confirming that by breaking up S–S bridges, DTT partly restituted the amplitude of the α,β-meATP current. DTT acted in an identical manner when rP2X3 (K201C/V274C) was transfected together with wild-type (wt) ASIC3 into CHO cells. Because Cys mutations at the neighboring amino acid residue of the rP2X3R (I200C/V274C) had no comparable effect, it was concluded that disulfide bridges can be generated only at specific sites within the receptor structure, if two amino acids are near enough ( ∼ 4.6 Ǻ) to allow the spontaneous constitution of an inter-subunit link. Hence, in a first approach it can be concluded that an unrestricted flexibility of the binding pouch of the P2X3R is a prerequisite for its interaction with ASIC3. 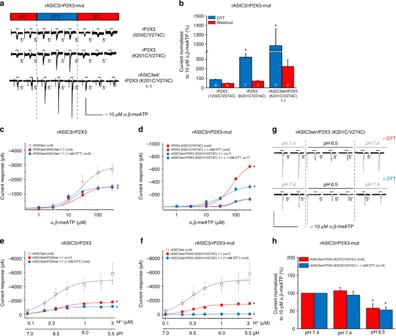Fig. 6 Effects of gate-inhibitory mutations in rP2X3Rs on rASIC3/rP2X3R function. Whole-cell patch-clamp recordings at a holding potential of −65 mV.a,bAnalysis of rP2X3 double cysteine mutants with disulfide trapping. CHO cells were transfected with the cysteine mutants rP2X3 (I200C/V274C), rP2X3 (K201C/V274C) or co-transfected with rASIC3wt and rP2X3 (K201C/V274C) in a 1:1 ratio.aCurrent traces induced by α,β-meATP (10 µM) applied repeatedly for 2 s with 5 min intervals before, during and after the co-application of ditiothreitol (DTT; 1 mM).bPercentage changes of α,β-meATP-induced current responses were calculated with respect to the mean of the second and third currents during DTT application. Means ± S.E.M. of the indicated number of experiments. *P< 0.05; statistically significant difference between the current amplitudes during and after DTT application (Student’st-test).c–fConcentration–response curves for protons and α,β-meATP in CHO cells co-transfected with the indicated receptors.cEffect of α,β-meATP (0.3–300 µM) on rP2X3Rwt, and rASIC3wt/rP2X3Rwt in the absence or presence of DTT.dEffect of α,β-meATP on rP2X3R (K201C/V274C) and rASIC3/rP2X3R (K201C/V274C) in the absence or presence of DTT.eEffect of protons (pH 7.0–5.5) on rASIC3wt and rASIC3wt/rP2X3Rwt in the absence or presence of DTT.fEffect of protons (pH 7.0–5.5) on rASIC3wt and rASIC3wt/rP2X3R (K201C/V274C) in the absence or presence of DTT. Means ± S.E.M. of the indicated number of experiments. *P<  0.05; statistically significant difference of theImeanvalues at the highest agonist concentration from the rP2X3Rwt and rASIC3wt curves, respectively (one-way ANOVA followed by the Holm–Sidak test).gInteraction between rASIC3wt and rP2X3R (K201C/V274C) in the absence and presence of DTT. Currents were elicited by α,β-meATP (10 µM) for 2 s with 5 min intervals before, during and after the pH shift from 7.4 to 6.5.hPercentage changes of α,β-meATP-induced current responses were calculated with respect to the second current before the pH shift. Means ± S.E.M. of the indicated number of experiments. *P< 0.05; statistically significant difference between the current amplitudes before and after the pH shift from 7.4 to 6.5 (Student’st-test). The scale labels for the vertical bars were 200 pA (a,g). The scale labels for the horizontal bars were 20 s (a) and 50 s (g) Fig. 6 Effects of gate-inhibitory mutations in rP2X3Rs on rASIC3/rP2X3R function. Whole-cell patch-clamp recordings at a holding potential of −65 mV. a , b Analysis of rP2X3 double cysteine mutants with disulfide trapping. CHO cells were transfected with the cysteine mutants rP2X3 (I200C/V274C), rP2X3 (K201C/V274C) or co-transfected with rASIC3wt and rP2X3 (K201C/V274C) in a 1:1 ratio. a Current traces induced by α,β-meATP (10 µM) applied repeatedly for 2 s with 5 min intervals before, during and after the co-application of ditiothreitol (DTT; 1 mM). b Percentage changes of α,β-meATP-induced current responses were calculated with respect to the mean of the second and third currents during DTT application. 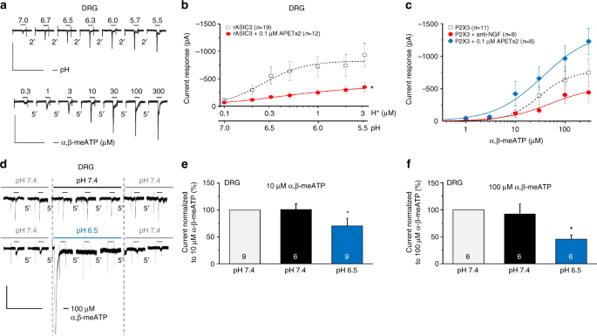Fig. 7 Electrophysiological interaction of native ASIC3 and P2X3Rs in rat DRG neurons. Whole-cell patch-clamp recordings at a holding potential of −65 mV. Rat cultured DRG neurons were used in all panels. Increasing concentrations of protons (pH 7.0–5.5) (a, upper panel) or α,β-meATP (0.3–300 µM) (a, lower panel) were applied in the presence of 10 µM capsazepine for 2 s with 2 min or 5 min intervals, respectively. DRG neurons were treated with APETx2 (0.1 µM;b,c) or anti-NGF (6 µg/ml for 24 h;c) while constructing concentration–response curves for protons or α,β-meATP. Means ± S.E.M. of the indicated number of experiments. *P< 0.05; statistically significant difference between theImeanvalues at the highest agonist concentrations (one-way ANOVA followed by the Hom–Sidak test).dCurrent responses were elicited by repeated applications of α,β-meATP (10 µM) for 2 s with 5 min intervals before, during and after the pH shift from 7.4 to 6.5; representative tracings. The peak of the proton-induced current was retouched in the lower panel of (d). Percentage changes of α,β-meATP-induced current responses at 10 µM (e) or 100 µM (f) were calculated with respect to the second current amplitude before the pH shift from 7.4 to 6.5. Means ± S.E.M. of the indicated number of experiments. *P< 0.05; statistically significant difference between the current amplitudes before and after the pH shift from 7.4 to 6.5 (one-way ANOVA followed by the Bonferroni test). The scale labels for the vertical bars were 500 pA (a) and 200 pA (b). The scale labels for the horizontal bars were 20 s (a) and 50 s (d) Means ± S.E.M. of the indicated number of experiments. * P < 0.05; statistically significant difference between the current amplitudes during and after DTT application (Student’s t -test). c – f Concentration–response curves for protons and α,β-meATP in CHO cells co-transfected with the indicated receptors. c Effect of α,β-meATP (0.3–300 µM) on rP2X3Rwt, and rASIC3wt/rP2X3Rwt in the absence or presence of DTT. d Effect of α,β-meATP on rP2X3R (K201C/V274C) and rASIC3/rP2X3R (K201C/V274C) in the absence or presence of DTT. e Effect of protons (pH 7.0–5.5) on rASIC3wt and rASIC3wt/rP2X3Rwt in the absence or presence of DTT. f Effect of protons (pH 7.0–5.5) on rASIC3wt and rASIC3wt/rP2X3R (K201C/V274C) in the absence or presence of DTT. Means ± S.E.M. of the indicated number of experiments. * P <  0.05; statistically significant difference of the I mean values at the highest agonist concentration from the rP2X3Rwt and rASIC3wt curves, respectively (one-way ANOVA followed by the Holm–Sidak test). g Interaction between rASIC3wt and rP2X3R (K201C/V274C) in the absence and presence of DTT. Currents were elicited by α,β-meATP (10 µM) for 2 s with 5 min intervals before, during and after the pH shift from 7.4 to 6.5. h Percentage changes of α,β-meATP-induced current responses were calculated with respect to the second current before the pH shift. Means ± S.E.M. of the indicated number of experiments. * P < 0.05; statistically significant difference between the current amplitudes before and after the pH shift from 7.4 to 6.5 (Student’s t -test). The scale labels for the vertical bars were 200 pA ( a , g ). The scale labels for the horizontal bars were 20 s ( a ) and 50 s ( g ) Full size image Of course, these considerations are valid only if DTT does not alter the current responses to α,β-meATP through wt P2X3Rs [27] or wt ASIC3/P2X3Rs (Fig. 6c ). Moreover, concentration–response curves for α,β-meATP obtained at cells transfected with Cys-mutated rP2X3 either alone or together with wt rASIC3 confirmed the data obtained with single concentrations of α,β-meATP (compare Fig. 6b with Fig. 6d ). There was a different situation, when the effect of protons was tested on CHO-rASIC3/rP2X3Rs or CHO-rASIC3/rP2X3R-mut cells. Co-transfection of rASIC3 with wt or mutant rP2X3Rs equally yielded lower maxima of the pH–current response curves in comparison with those obtained in CHO cells transfected with rASIC3 alone (Fig. 6e, f ). Contrary to our expectations, DTT did not restitute the effect of protons in the cells transfected with the two wt receptors, but strongly inhibited the effect of acidification, when transfection was with rASIC3/rP2X3 (K201C/V274C). In spite of this massive inhibitory effect, DTT did not prevent the depression of the response to a single concentration of α,β-meATP in interaction experiments (Fig. 6g, h ). Thus, DTT application has led to structural rearrangement of Cys-mutated rASIC3/rP2X3-mut receptors by breaking up the newly generated S–S bonds resulting in insensitivity to protons. However, this procedure did not interfere with the effect of α,β-meATP in interaction experiments. Interaction between the two native receptors The next question to be answered was to which extent ASIC3 and P2X3Rs co-exist in rat DRG neurons. Moderate acidification (pH 7.0–5.5) in the presence of the TRPV1 receptor antagonist capsazepine (10 µM) produced pH-dependent, rapidly desensitizing inward currents which were inhibited by the selective ASIC3 antagonist APETx2 (0.1 µM) (Fig. 7a , upper panel, Fig. 7b ) [28] . α,β-meATP (0.3–300 µM) also induced concentration-dependent inward currents which were similar in shape to those evoked by pH changes (Fig. 7a , lower panel). The amplitudes of the current responses to α,β-meATP were not altered either after the application of APETx2 (0.1 µM) or after incubation with anti-nerve growth factor antibody (anti-NGF, 6 µg/ml for 24 h) (Fig. 7c ). Nonetheless, the tendency of the concentration–response curves to change was such that APETx2 appeared to facilitate while anti-NGF appeared to depress the effects of α,β-meATP. Fig. 7 Electrophysiological interaction of native ASIC3 and P2X3Rs in rat DRG neurons. Whole-cell patch-clamp recordings at a holding potential of −65 mV. Rat cultured DRG neurons were used in all panels. Increasing concentrations of protons (pH 7.0–5.5) ( a , upper panel) or α,β-meATP (0.3–300 µM) ( a , lower panel) were applied in the presence of 10 µM capsazepine for 2 s with 2 min or 5 min intervals, respectively. DRG neurons were treated with APETx2 (0.1 µM; b , c ) or anti-NGF (6 µg/ml for 24 h; c ) while constructing concentration–response curves for protons or α,β-meATP. Means ± S.E.M. of the indicated number of experiments. * P < 0.05; statistically significant difference between the I mean values at the highest agonist concentrations (one-way ANOVA followed by the Hom–Sidak test). 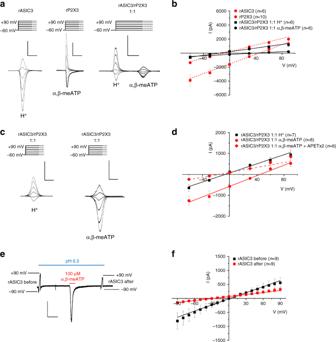d Current responses were elicited by repeated applications of α,β-meATP (10 µM) for 2 s with 5 min intervals before, during and after the pH shift from 7.4 to 6.5; representative tracings. The peak of the proton-induced current was retouched in the lower panel of ( d ). Fig. 5 Switch of reversal potentials between co-expressed rASIC3 and rP2X3Rs in CHO cells. Whole-cell patch-clamp recordings at a holding potential of −65 mV.aCurrent traces induced by protons (pH 6.5) and α,β-meATP (10 µM) applied individually onto CHO-rASIC3 (left panel) and CHO-rP2X3R cells (middle panel) or successively onto CHO-rASIC3/P2X3 cells (right panel). Agonist application was at holding potentials which increased stepwise from −60 to + 90 mV in 30 mV increments. Current–voltage relationships were constructed from recordings similar to those shown in (a) in order to determine the reversal potentials (Erev) (b). Means ± S.E.M. of the indicated number of experiments.cMeasurement ofErevof protons (left panel) and of α,β-meATP (right panel) by a similar protocol as shown in (a) on separate populations of CHO-rASIC3/rP2X3R cells. Under these conditions, theErevvalues of these two agonists were interchanged. Current–voltage relationships constructed from recordings similar to those shown in (c) in order to determine theErev(d). Means ± S.E.M. of the indicated number of experiments. Blockade of ASIC3 channel activity by the selective antagonist APETx2 (0.1 µM) shifted theErevof α,β-meATP back near to its original value of around 0 mV.eIn CHO-rASIC3/rP2X3R cells, ramps of 200 mV duration (−90 to  +90 mV) were delivered at a holding potential of −65 mV to determine theErevof ASIC3 after a drop of the normal pH from 7.4 to 6.5. Then, a high concentration of α,β-meATP (100 µM) was applied in order to change the distribution of extra- and intracellular ions. Eventually, theErevwas re-determined after washing out α,β-meATP. Original tracing; large capacitive artifacts at the beginning and end of the ramp-induced currents were retouched.fCurrent–voltage curves were constructed from the indicated number of experiments similar to that shown in (e). The scale labels for the vertical bars were 2 nA (a, left panel), 1 nA (a, middle and right panels), 1 nA (c) and 500 pA (e). The scale labels for the horizontal bars were 1 s (a,c) and 2 s (e) Percentage changes of α,β-meATP-induced current responses at 10 µM ( e ) or 100 µM ( f ) were calculated with respect to the second current amplitude before the pH shift from 7.4 to 6.5. Means ± S.E.M. of the indicated number of experiments. * P < 0.05; statistically significant difference between the current amplitudes before and after the pH shift from 7.4 to 6.5 (one-way ANOVA followed by the Bonferroni test). The scale labels for the vertical bars were 500 pA ( a ) and 200 pA ( b ). The scale labels for the horizontal bars were 20 s ( a ) and 50 s ( d ) Full size image Further, native rASIC3 and rP2X3R-mediated current responses in DRGs cultured in the presence of NGF showed the same type of interaction between the two receptor channels as observed between their recombinant counterparts (Fig. 7d–f ). An important difference, however, was that an increase in the concentration of α,β-meATP from 10 to 100 µM increased rather than decreased the extent of the proton-induced inhibition imposed upon rP2X3Rs. This may be due to the pH-induced stimulation of other receptor types not present in CHO cells, which might modulate the ASIC3–P2X3R interaction. The above-mentioned concentration of anti-NGF antibodies was sufficient to neutralize endogenous NGF [29] . To investigate the role of NGF in the expression of ASIC3 and P2X3R immunoreactivities in our DRG cultures, we used cells grown either in the absence or in the presence of NGF. Most cells exhibited ASIC3 and P2X3R immunoreactivity under either condition; however, this staining was much weaker in the absence of NGF (Fig. 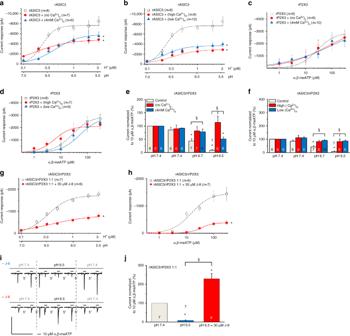8a ). Thus, NGF, which is supposed to be a mediator of neuroinflammation, increased the expression but not the function of ASIC3 and P2X3Rs (see ref. [29] ). Fig. 4 Changes in the Ca2+concentration modify rASIC3 and rP2X3R currents in CHO cells. Whole-cell patch-clamp recordings at a holding potential of −65 mV.a,bConcentration–response curves for protons in CHO cells transfected with rASIC3.aInhibitory effect of an increase or decrease of the Ca2+concentration in the external medium ([Ca2+]o).bInhibitory effect of an increase or decrease of the free Ca2+concentration in the patch pipette solution ([Ca2+]i).c,dConcentration-response curves for α,β-meATP in CHO cells transfected with rP2X3.cNo effect of changes in [Ca2+]o.dNo effect of changes in [Ca2+]i. Means ± S.E.M. of the indicated number of experiments. *P< 0.05; statistically significant difference of theImeanvalues at the highest agonist concentration (one-way ANOVA followed by the Holm–Sidak test).e,fCHO cells transfected with both rASIC3 and rP2X3 in a 1:1 ratio. Modulation of the unilateral interaction between rASIC3 and rP2X3Rs, by changes in [Ca2+]o(e) and [Ca2+]i(f); the experimental protocol is identical to that shown in Fig.2a. *P< 0.05; statistically significant difference from the current amplitudes measured in normal extra- and intracellular Ca2+.§P< 0.05; statistically significant difference between currents at pH 6.7 or 6.5 at different Ca2+concentrations (one-way ANOVA followed by the Bonferroni test). Concentration–response relationships for protons (g) and α,β-meATP (h) in CHO-rASIC3/rP2X3R cells, in the absence and presence of J-8 (30 µM). Means ± S.E.M. of the indicated number of experiments. *P< 0.05; statistically significant difference between theImeanvalues at the highest agonist concentration (Student’st-test).iPotentiation of the α,β-meATP (30 µM) current by co-application with a J-8 (30 µM)-containing, low pH (6.5) external medium, but inhibition in the absence of J-8 by acidification; representative tracings.jPercentage changes of α,β-meATP-induced current responses were calculated with respect to the second current amplitude before the pH shift. Means ± S.E.M. of the indicated number of experiments. *P< 0.05; statistically significant difference between the current amplitudes before and after the pH shift from 7.4 to 6.5 in the presence of J-8.§P< 0.05; statistically significant difference between current amplitudes at pH 6.5 in the presence or absence of J-8 (Mann–Whitney test). The scale labels for the vertical and horizontal bars in (i) were 1 nA and 50 s, respectively This may indicate that the ‘cognate’ ASIC3/P2X3R is mainly involved in inflammatory pain accompanied by a drop in pH. Fig. 8 Immunoreactivity, co-immunoprecipitation and membrane expression of rASIC3 and rP2X3Rs in rat DRG neurons. a ASIC3 and P2X3R immunoreactivities in rat DRG neurons cultured in the presence (upper panel) or absence (lower panel) of nerve growth factor (NGF). Hoechst (Hoe) was used to stain the cell nuclei. b Examples of immunoprecipitation (IP) of DTSSP-treated extracts of primary sensory neurons with P2X3 antibodies revealed in western blots (WB) with anti-ASIC3 antibodies. Incubation of neuronal cultures at pH 6.8 or 7.5 has no effect. ASIC3 signal is not found after immunoprecipitation with unrelated antibodies (IgG). Input ASIC3 and P2X3 contents in total extracts are also shown. β-Actin is used as gel loading control. c Examples of immunoprecipitation of P2X3 receptors (P2X3, upper panel) with ASIC3 channels in control conditions (scramble) and after P2X3 receptor silencing (siP2X3). No P2X3/ASIC3 signal was found after siP2X3 treatment. Western blot with anti-ASIC1 or anti-ASIC2 antibodies gave no signal. Pull down with unrelated antibody (IgG) gave no signal. Quality of input lysates and equal gel loading is shown (lower panel, total lysates). d Surface expression of P2X3Rs. Example of membrane protein biotinylation experiments in CHO cells transfected with plasmids encoding for ASIC3 alone or ASIC3 plus P2X3Rs (upper panel, surface). Quality of total protein extracts and controls for equal gel loading are also shown (bottom panel, total lysates). The scale labels in the right upper and lower panels of ( a ) were 20 µm Full size image Eventually, to test the supposed spatial vicinity of ASIC3 and P2X3Rs, a series of immunoprecipitation and western blot experiments were performed (Fig. 8b, c ). Measurements in rat DRG cultures pre-treated with the protein crosslinker DTSSP (2 mM; Fig. 8b ) demonstrated the existence of an ASIC3/P2X3R complex with a signal (59 kDa), not detectable in the control lane. The application of the TRPV1 antagonist capsazepine (10 µM, 30 min pre-incubation) had no influence on the results. To confirm P2X3/ASIC3 interaction in rat DRG samples, we silenced endogenous P2X3 with siP2X3, and performed pull-down experiments with anti-P2X3 antibodies and western blot with anti-ASIC1, ASIC2 or ASIC3 (Fig. 8c ). These experiments showed the exclusion of ASIC1 and ASIC2 from the P2X3 molecular complex and lack of ASIC3 pull-down after P2X3R silencing (Fig. 8c , upper panel). Notably, ASIC3 expression did not change after siP2X3 (Fig. 8c , lower panel). Lack of ASIC1/P2X3R interaction in DRG neurons, in spite of opposite electrophysiological data obtained with recombinant receptors in transfected CHO cells, may be due to their non-physiological over-expression in the latter cell type. Membrane protein biotinylation of recombinant ASIC3/P2X3 plasmids confirmed that the expression of ASIC3 at the cell surface (labeled by the membrane-impermeable biotin) was not influenced by the simultaneous expression of P2X3Rs (Fig. 8d ). For the uncropped images of the cropped displayed plots shown in Fig. 8b–d , see the Suppl. Fig. 3a–c . Interaction between the two receptors in oocytes Xenopus laevis oocytes offer the unique advantage that an exactly defined molar ratio of two distinct cRNAs can be delivered by microinjection into every cell. In oocytes expressing the His-rP2X3-StrepII receptor (rP2X3R) only, acidification to pH 6.5 did not alter the current amplitudes induced by α,β-meATP (3 µM) (Suppl. Fig. 2a, c , left panel). By contrast, in oocytes co-expressing His 8 -rASIC3-EGFP and His-rP2X3-StrepII receptors (rASIC3/rP2X3R) the effect of α,β-meATP (3 μM) was markedly inhibited by the same change in pH (Suppl. Fig. 2b, c , right panel). Essentially the same findings were obtained when a higher concentration of α,β-meATP (10 µM) was used (Suppl. Fig. 2d , left panel), although the inhibition caused by protons (pH 6.5) was less pronounced in rASIC3/rP2X3R cells (Suppl. Fig. 2d , right panel). Hence, rASIC3 and rP2X3Rs showed the same type of interaction irrespective of the expression systems utilized. To analyze whether rASIC3 and rP2X3 form oligomeric complexes incorporating both subunits, we co-expressed His-rP2X3-StrepII together with His 8 -rASIC3-EGFP as bait and prey proteins, respectively. The plasma membrane-bound pool of both subunits was labeled with the membrane-impermeant fluorescence dye Cy5-NHS ester. The non-StrepII-tagged His-rASIC3-EGFP subunits did not bind to the Strep-Tactin resin (Fig. 9a , lanes 1 and 2). Sodium dodecyl sulfate–polyacrylamide gel electrophoresis (SDS-PAGE) revealed an apparent molecular mass of the His-rASIC3-EGFP subunit of ~75 kDa (as referred to the mass marker) (Fig. 9a , lanes 3 and 4). The His-rP2X3-StrepII subunit was purified in its plasma membrane-bound form, as visualized by the red (Cy5) fluorescent ~54 kDa polypeptide (Fig. 9a , lanes 13–16). Following co-expression of both subunits, the His-rASIC3-EGFP subunit was co-purified by Strep-Tactin chromatography (Fig. 9a , lanes 7, 8 and 11, 12). Fig. 9 Plasma membrane expression and oligomeric assembly of rASIC3 and rP2X3R subunits in oocytes. For biochemical analysis, Xenopus (X.) laevis oocytes expressing the indicated proteins were surface labeled with the membrane-impermeant fluorescent Cy5 dye before protein purification. The indicated proteins were purified under non-denaturing conditions from X. laevis oocytes by Ni 2+ -NTA chromatography or Strep-Tactin chromatography, as indicated, resolved by SDS-PAGE ( a ) or BN-PAGE ( b ), and visualized by Typhoon fluorescence scanning. a Overlay of the Cy5-labeled surface form (red) of the His-rASIC3-EGFP and His-rP2X3-StrepII protomers and the GFP fluorescence (green) of the His-rASIC3-EGFP protomer. The positions of molecular mass markers (in kDa) are shown on the left. b Overlay of GFP and Cy5 fluorescence of the homomeric His-rASIC3-EGFP (lanes 1–4) and homotrimeric His-rP2X3-StrepII (lanes 15–18) and the co-expressed His-rASIC3-EGFP and His-rP2X3-StrepII receptor subunits (lanes 5–14) in their native or partial SDS-denatured forms isolated by Ni 2+ -NTA (lanes 3–6, 10, 11, 15, 16) or Strep-Tactin (lanes 7–9, 12–14, 17, 18) chromatography as indicated. Co-expression of rASIC3 and rP2X3 (lanes 5–14) originates from the co-injection of the His-rASIC3-EGFP and His-rP2X3-StrepII subunit in cRNA ratios as indicated. The number of protomers included in the respective bands are exemplarily indicated. The inset shows the indicated section of the gel with enhanced GFP fluorescence to enable the visibility of the ASIC3 trimer. The schematics and labeling on the left or right margins indicate the numbers of rASIC3 or rP2X3 protomers incorporated in the respective trimeric (bold) or dimeric or monomeric protein band of the rASIC3 or rP2X3 receptor complexes, respectively Full size image The same samples as in Fig. 9a were also resolved in the non-denatured and partially SDS-denatured state by blue native-polyacrylamide gel electrophoresis (BN-PAGE; Fig. 9b ). The homotrimeric state of the His-rP2X3-StrepII receptor was verified by partial denaturing of the native receptor complexes, resulting in the appearance of homodimers and prominent monomers (Fig. 9b , lanes 15–18). A small fraction of the non-denatured His-rP2X3-StrepII receptor migrated as higher-order assemblies consisting of dimers of trimers (Fig. 9b , e.g., lane 15), consistent with previous reports [30] , [31] . The His-rASIC3-EGFP receptor complex is significantly larger than the His 6 -rP2X3-StrepII receptor due to the per se larger mass of the rASIC3 subunit and the fused 27 kDa enhanced green fluorescent protein (EGFP) moiety. The non-denatured His-rASIC3-EGFP receptor migrates as a ladder of bands. Using the defined His-rP2X3-StrepII oligomers as mass markers consisting of one to six 55 kDa protomers, the His-rASIC3-EGFP receptor was determined to primarily migrate as monomers, dimers and trimers of protomers of ~75 kDa (Fig. 9b , lane 3). Partial denaturing dissolved the higher-order aggregates in favor of dimers and monomers (Fig. 9b , lane 4). BN-PAGE analysis (Fig. 9b ) of the non-denatured proteins purified by Strep-Tactin chromatography revealed the plasma membrane-bound His-rP2X3-StrepII as a homotrimer of 165 kDa irrespective of whether the His-rP2X3-StrepII was expressed alone (lane 17) or together with various amounts of co-expressed His-rASIC3-EGFP (lanes 7 and 12). Any co-assembly with one or two copies of His-rASIC3-EGFP should result in the appearance of a heterotrimer of significantly increased mass as compared to the His-rP2X3-StrepII homotrimer. Such a mass shift was evidently not observed. The incorporation of one or two His-rASIC3-EGFP copies would be further indicated by EGFP fluorescence, which was also not observed. However, there is evidence for the co-purification of His-rASIC3-EGFP homotrimers (weakly visible in lane 7, see inset) that dissociated into His-rASIC3-EGFP monomers when partially denatured with SDS (lanes 8 and 9; also visible in lanes 13 and 14 following injection of a fourfold lower amount of His-rASIC3-EGFP cRNA). These results can be best reconciled with the view that rASIC3 and rP2X3R form a complex of two separate homotrimers rather than to form heterooligomers co-assembled of both rASIC3 and rP2X3R subunits. Hyperalgesia induced by acidification and purinergic stimulation The next set of experiments explored the interaction of mechanical hyperalgesia induced by local acidification (pH 7.0, 6.5) and α,β-meATP (50 nmol) in vivo. Intraplantar (i.pl.) administration of pH-adjusted phosphate-buffered saline (PBS) solution decreased the paw withdrawal threshold (PWT) values in a pH-dependent manner, indicating the development of acidification-induced mechanical hyperalgesia, while the administration of pH 7.4 PBS caused negligible change from the baseline PWT at any time point (Fig. 10a ). The mechanical hypersensitivity to i.pl. pH-adjusted PBS recovered at the 4-h post-injection time point (Fig. 10a ). Fig. 10 The effect of normal and pH-adjusted PBS solution and α,β-meATP on mechanical hyperalgesia in rats. a Time–response curves of the effect of intraplantar (i.pl.) phosphate-buffered saline (PBS) or α,β-meATP (50 nmol) dissolved in PBS injected into the right hind paw at a volume of 100 µl/paw on the baseline mechanical paw withdrawal threshold (PWT). Each point represents mean ± S.E.M. of the PWT in pressure as a percentage of baseline % applied to the hind paw before (pre) and after PBS/α,β-meATP administration, obtained from the indicated number of rats. α,β-meATP decreased PWT both pH and time dependently post injection (repeated measures ANOVA time × treatment effect F 1,38 = 1.760, P < 0.00001). 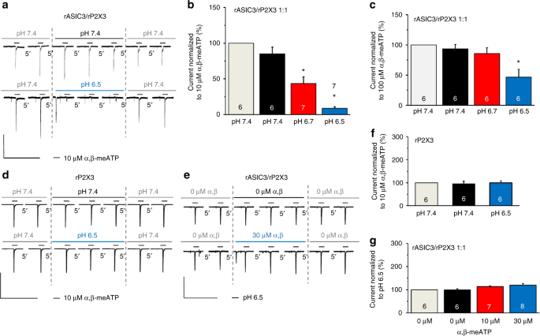The changes from baseline PWT were at pH 7.4, 16.5% ( P = 0.0026, n = 6), at pH 7.0, 25.6% ( P = 0.001, n = 6), at pH 6.5, 33.3% ( P < 0.001, n = 6, one-way ANOVA followed by the Dunnett test) at 1 h. For the sake of clarity, statistical significance is not indicated in the figure. b Dose-dependent effect of α,β-meATP on mechanical hyperalgesia at pH 7.0. § P < 0.05; statistically significant difference vs. baseline; * P < 0.05; statistically significant difference vs. PBS. Results were analyzed by repeated measures ANOVA, followed by Neuman–Keuls test, n = 6–10 animals per group. Fig. 2 Interaction between rASIC3 and rP2X3Rs after their transfection into CHO cells. CHO cells were transfected with rASIC3 and rP2X3Rs in a 1:1 ratio or transfected only with rP2X3R as indicated. Whole-cell patch-clamp recordings at a holding potential of −65 mV.a–cInteraction between rASIC3 and rP2X3Rs on their sequential activation by agonists. Current responses were elicited by α,β-meATP (10 or 100 µM) for 2 s with 5 min intervals before, during and after a shift in pH from 7.4 to 6.7 or 6.5. The reproducibility of the responses to α,β-meATP after changing to a solution with the same pH of 7.4 is also shown.d,fNo effect of protons on rP2X3Rs. Current responses were elicited by α,β-meATP (10 µM) for 2 s with 5 min intervals before, during and after a shift in pH from 7.4 to 6.5.e,gNo effect of α,β-meATP (10 and 30 µM) on the proton-induced inward current on the sequential activation of rP2X3 and rASIC3Rs. Stable responses to pH 6.5 in the absence of α,β-meATP is also shown. Percentage changes of α,β-meATP (10 and 100 µM)-induced current responses were calculated with respect to the second current before the pH shift to 6.7 or 6.5 (b,c,f). Percentage changes of proton (pH 6.5)-induced current responses were calculated with respect to the second current amplitude before the application of α,β-meATP (0, 10 and 30 µM) (g). Means ± S.E.M. of the indicated number of experiments. *P< 0.05; statistically significant difference between the current amplitudes before and after the long-lasting shift in pH or the long-lasting presence of α,β-meATP (one-way ANOVA followed by the Bonferroni test). The scale labels for the vertical bars were 500 pA (a) and 2 nA (d,e). The scale labels for the horizontal bars were 50 s (a,d,e) c The effect of acidification on α,β-meATP-induced hyperalgesia. PWT values were normalized to the response obtained by 50 mM α,β-meATP at pH 7.4. * P < 0.05; statistically significant difference from the 100%. Results were analyzed by one-way ANOVA followed by Tukey test, n = 6 animals per group Full size image Next we examined the effect of α,β-meATP (50 and 100 nmol) at pH 7.0 which also induced mechanical hyperalgesia in a dose- and time-dependent manner, when compared to baseline values, or to the administration of PBS alone (Fig. 10b ). Finally, we tested the effect of the lower, 50 nmol dose of α,β-meATP on three different pH levels (Fig. 10a, c ). We found that at lower pH the hyperalgesia evoked by α,β-meATP was significantly facilitated and administration of pH-adjusted α,β-meATP elicited significant difference from the baseline PWT at 1 h (Fig. 10c ). The facilitation of the hyperalgesic effect of α,β-meATP by pH changes from 7.4 to 7.0 and 6.5 are in agreement with the involvement of an rASIC3/rP2X3R in the sensation of pain. A wealth of data obtained with electrophysiology, co-immunoprecipitation, fluorescence resonance energy transfer analysis and biochemistry demonstrates that different recombinant and native ASIC subunits can form heteromeric channels (e.g., 1a/2a) [32] , [33] . Based on a systematic biochemical analysis of P2X subunits over-expressed in HEK cells, it was reported that all subunits can hetero-oligomerize with a particular partner, with the exception of P2X7 [30] , [34] , [35] . 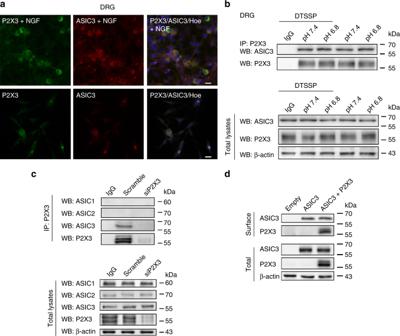Fig. 8 Immunoreactivity, co-immunoprecipitation and membrane expression of rASIC3 and rP2X3Rs in rat DRG neurons.aASIC3 and P2X3R immunoreactivities in rat DRG neurons cultured in the presence (upper panel) or absence (lower panel) of nerve growth factor (NGF). Hoechst (Hoe) was used to stain the cell nuclei.bExamples of immunoprecipitation (IP) of DTSSP-treated extracts of primary sensory neurons with P2X3 antibodies revealed in western blots (WB) with anti-ASIC3 antibodies. Incubation of neuronal cultures at pH 6.8 or 7.5 has no effect. ASIC3 signal is not found after immunoprecipitation with unrelated antibodies (IgG). Input ASIC3 and P2X3 contents in total extracts are also shown. β-Actin is used as gel loading control.cExamples of immunoprecipitation of P2X3 receptors (P2X3, upper panel) with ASIC3 channels in control conditions (scramble) and after P2X3 receptor silencing (siP2X3). No P2X3/ASIC3 signal was found after siP2X3 treatment. Western blot with anti-ASIC1 or anti-ASIC2 antibodies gave no signal. Pull down with unrelated antibody (IgG) gave no signal. Quality of input lysates and equal gel loading is shown (lower panel, total lysates).dSurface expression of P2X3Rs. Example of membrane protein biotinylation experiments in CHO cells transfected with plasmids encoding for ASIC3 alone or ASIC3 plus P2X3Rs (upper panel, surface). Quality of total protein extracts and controls for equal gel loading are also shown (bottom panel, total lysates). The scale labels in the right upper and lower panels of (a) were 20 µm However, only P2X2/3Rs (sensory ganglia) [10] , [36] and P2X1/5Rs (astrocytes) [37] , [38] were shown to occur under native conditions, whereas P2X1/2, P2X1/4, P2X2/6 and P2X4/6Rs were hitherto not identified in mammalian tissues. The aim of this study was to decide whether the two structurally related subunits ASIC3 and P2X3 are able to form a heterotrimeric receptor or whether they assemble into two separate channels. Our data strongly suggest the existence of a ‘cognate receptor’ which, in contrast to other P2X3R/Cys-loop-R associations (see Introduction), contains proteins interacting with each other in an unusual manner. It has to be mentioned at this stage that whereas we report that the activation of ASIC3 by protons inhibits P2X3R-mediated effects, the activation of a P2X5R by ATP has been found to potentiate the effect of protons on ASIC3 [39] . There are many additional differences between the ASIC3/P2X3R and P2X5R/ASIC3 interactions, such as the sensitivity to intracellular Ca 2+ , reversibility of the inhibition after removal of the respective agonists, limitation to a certain subtype of DRG neurons, switch of the ionic permeability between the two receptor channels, etc., all characteristics of the ASIC3/P2X3R interaction only. Thus, we conclude that two fundamentally different reactions take place, establishing a forward and backward connection between the acid and ATP-responsive sensory elements. It is interesting to note that the unilateral interaction between rASIC3 and rP2X3Rs depends on the stimulation of the proton-binding site, because activation of the non-proton-binding site with GMQ [23] inhibited the α,β-meATP-induced current response by another mechanism. Then, we concentrated ourselves on the situation occurring when instead of rASIC3, rASIC1a or rASIC2a were available as possible interaction partners for rP2X3Rs. The pH 50 value of rASIC1a is similar to but that of rASIC2a is considerably lower than that of rASIC3 [7] , [40] . The distribution of these channels in the nervous system also differs in that ASIC3 is mostly peripherally located, while ASIC1a and ASIC2a exist in both the peripheral nervous system and central nervous system. Interestingly, the association with rP2X3Rs depressed the I mean values of both rASIC1a and -2a, although only rASIC1a was able to depress the rP2X3R currents in analogy with ASIC3. rASIC1 and rASIC3 currents are induced by moderate acidification in rat DRG neurons, whereas rASIC2 and transient receptor potential vanilloid 1 (rTRPV1) currents have been described to activate at lower pH values [41] , [42] . Of various ASICs only rASIC3 shows biphasic desensitization kinetics with both a rapidly inactivating and a sustained component. The ‘a’ isoform of human (h) ASIC3 shares 84% sequence identity with rASIC3 and exhibits similar desensitization kinetics [22] . We used in our experiments the ‘b’ isoform of hASIC3 and showed that it required more acidic pH for activation than its rat ortholog. Next, we studied the possible involvement of Ca 2+ in the interaction between rASIC3 and rP2X3Rs. It has been reported that protons open ASIC3 by accelerating the release of Ca 2+ from a high-affinity binding site on the extracellular side of the pore [43] , [44] . P2X3Rs are regulated by an intracellular calcium/calmodulin-dependent serine protein kinase (CASK) which phosphorylates and in consequence upregulates this receptor, resulting in larger current responses to agonists [45] . P2X3Rs can be phosphorylated by an ecto-protein kinase as well [46] . In partial agreement with these results we found that changes in both intra- and extracellular Ca 2+ concentrations inhibited rASIC3- but not rP2X3R-mediated currents. Moreover, changes of [Ca 2+ ] o or [Ca 2+ ] i into either direction blocked the rASIC3/rP2X3R interaction. The calmodulin antagonist J-8 depressed the effects of both protons and α,β-meATP in CHO-rASIC3/rP2X3R cells and in addition turned the inhibitory interaction between the two receptor channels into potentiation. Thus, we identified Ca 2+ as a modulator subserving at least partially the interaction between rASIC3 and rP2X3Rs. Already at this stage we tentatively concluded that a ‘cognate’ rather than a heterotrimeric receptor has been constructed after co-transfecting the two receptors into CHO cells. Measurements of reversal potentials in CHO-ASIC3/P2X3R cells supported this idea by twofold evidence. (1) When protons and α,β-meATP were applied sequentially, the ASIC3 current had a reversal potential of around 0 mV (otherwise characteristic for P2X3R currents) and the P2X3R current displayed a reversal potential of somewhat below +65 mV (otherwise characteristic for ASIC3R currents). It appeared that a redistribution of cations between the intra- and extracellular space, due to the application of α,β-meATP, was not the cause of this phenomenon. Hence, the two ion channels appeared to switch their ionic permeabilities because of their intimate spacial relationship. (2) A similar switch of the ionic permeabilities was observed when in a series of experiments only protons were applied to CHO-ASIC3/P2X3R cells and in the other series only α,β-meATP. It was a regular observation that the current amplitudes through all ASICs investigated (rASIC3, rASIC1a, rASIC2a, hASIC3) became smaller when they were co-transfected together with P2X3Rs (rP2X3 or hP2X3). We considered it likely that a functional interaction of ASICs with the non-activated (closed-state) P2X3R is responsible for this effect. Of course, a further possibility is that P2X3Rs interfere with the assembly or trafficking of ASICs to the cell membrane and their subsequent insertion into it. However, our biochemical data from oocytes did not provide evidence for this assumption, although they revealed that co-expression of sASIC3/rP2X3R subunits in a 1:1 ratio slightly reduced the appearance of rP2X3R homotrimers at the cell surface. Further, membrane protein biotinylation of CHO cells transfected with ASIC3 and P2X3 plasmids confirmed that the expression of ASIC3 at the cell surface was not influenced by the simultaneous expression of P2X3Rs. Therefore, we set out to investigate whether the depression of the ASIC3 I max and/or the negative functional interaction between ASIC3 and P2X3Rs may be modified by the perturbed agonist binding pouch of rP2X3Rs or of its restricted conformational flexibility. Mutagenesis studies at homomeric P2XRs uniformly suggest that the negatively charged phosphate groups of ATP occupy some positively charged amino acids, specifically Lys or Arg [47] . The absolute requirement for Lys-63 and Lys-299 in P2X3Rs for agonist binding has been repeatedly confirmed by Ala replacement of these amino acids [25] , [48] and conforms with predictions made on the basis of the crystal structure of P2X3Rs [49] , [50] . Furthermore, the conformational flexibility of the three subunits of a P2XR is an indispensable prerequisite for channel opening; after the introduction of Cys residues at certain critical sites of the receptor channel, disulfide bonds are formed and the receptor becomes immobilized in one state of operation, resulting in a loss of functionality [27] , [51] , [52] . The K201C/V271C mutation of the P2X3R does not directly interfere with agonist binding and supposedly blocks the agonist-induced current via an interference with channel gating [27] . In the present work, dominant negative Ala-mutants of the rP2X3R component of the rASIC3/rP2X3R strongly depressed the I max of protons at wt ASIC3; however, the extent of this depression failed to surmount that exerted by wt P2X3Rs itself. Thus, the agonist binding site did not modify the rASIC3/rP2X3R function. Moreover, immobilizing Cys mutations also did not appear to alter the proton-induced current at rASIC3/rP2X3R. However, breaking up the inactivating disulfide bridges by DTT nearly abolished the function of the rASIC3/rP2X3R instead of rescuing its original activity. We hypothesize that this may be due to an altered conformational rearrangement of the individual subunit assembly in the ‘cognate’ receptor structure after DTT application. It was most important to confirm that native ASIC3/P2X3Rs in rat DRG neurons behave in a manner similar to the recombinant receptor assemblies. For this purpose we used rat DRG neurons cultured in the presence of NGF which is known to be an inflammatory modulator [53] . Most DRG neurons co-expressed rASIC3 with rP2X3Rs, as shown by means of immunohistochemistry and patch-clamp recordings. Both the intensity of the immunostaining for ASIC3 and P2X3Rs and the amplitude of the α,β-meATP-induced current responses critically depended on NGF; these current amplitudes were depressed but were not abolished by an anti-NGF antibody [29] . At a first glance, this finding is difficult to reconcile with the reported data showing that under in vivo conditions remarkably few DRG neurons ( ∼ 10%) co-express ASIC3 and P2X3Rs [54] . It can be argued that the difference between the in vivo and in vitro situation is due to the inevitable damage inflicted to the neurons by the preparation and culturing procedures. A particularly strong evidence for the involvement of ASIC3 in the proton-induced currents in rat DRGs was the inhibitory activity of the selective antagonist APETx2 [28] . In support of the current measurements, pull-down experiments with an anti-P2X3R-antibody demonstrated the close spatial vicinity of rASIC3, but not of ASIC1 or ASIC2, and P2X3Rs in DRG cells. Cutaneous hyperalgesia in rats was induced by the injection of both a low pH solvent and α,β-meATP into the hind paw. The effect of a stable dose of intraplantar α,β-meATP was pH-dependently potentiated, suggesting an additive instead of an inhibitory interaction between rASIC3 and rP2X3Rs already around pH 7.0, characteristic for the low activation threshold of these channels. However, it is noteworthy that the percentage algogenic effect of α,β-meATP increased in parallel with the enhancement of the external pH, just as it was observed in electrophysiological experiments with DRG neurons. It has been reported that ASIC3 mediates mechanical hyperalgesia associated with muscle inflammation [55] , [56] . The present experiments suggested that not only muscle but also other sensory afferents (e.g., skin) appear to be endowed with ASIC3, especially because in our electrophysiological experiments practically all cultured DRG neurons possessed proton-induced ion channels blocked by APETx2. Following co-expression of His-rASIC3-GFP and His-rP2X3-StrepII subunits in X. laevis oocytes, the His-rASIC3-GFP subunit could be co-isolated by Strep-Tactin chromatography in amounts that varied depending on the relative availability of rASIC3 and rP2X3 subunits. However, non-denaturing BN-PAGE analysis showed exclusively His-rP2X3-StrepII and His-rASIC3-GFP homotrimers, but no heteromeric assemblies containing both rASIC3-GFP and rP2X3 subunits. We did not extend our investigations to tranfected CHO cells, because previous work demonstrated an absolute comparability of results obtained by the biochemical analysis of P2X3R oligomerization and surface expression in X. laevis oocytes and HEK293 cells [25] , [26] , [27] , [48] . Moreover, electrophysiological recordings showed that the activation of rASIC3 depressed the rP2X3R currents in both CHO cells and oocytes in a similar manner. In conclusion, multiple evidence suggests that ASIC3 and P2X3Rs form a ‘cognate’ receptor, as supported by electrophysiology, immunohistochemistry, co-immunoprecipitation, biochemistry and pain measurement. 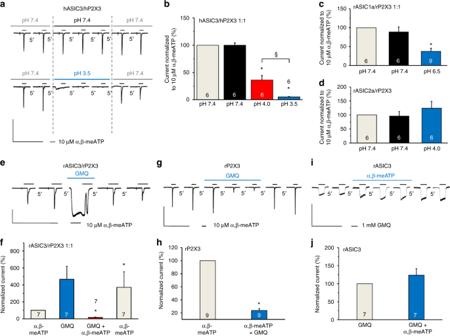Plasmid preparation and site-directed mutagenesis The rASIC3 cDNA subcloned into the plasmid pEGFP-C3 as well as the rASIC1a and -2a cDNAs were gifts from Eric Lingueglia (Université de Nice Sophia Antipolis, Valbonne, France). rP2X3 cDNA was a gift from Ye Yu (Institute of Neuroscience and State Key Laboratory of Neuroscience, Shanghai, China). The cDNA encoding for hASIC3b was kindly provided by Günther Schmalzing (RWTH Aachen University, Germany). The cDNAs were subcloned into the plasmid pIRES2-EGFP (all ASICs, except rASIC3) or pIRES2-RFP (P2X3), which were available from previous studies [26] . Primers used for mutagenesis were synthesized by MWG Biotech (Suppl. Fig. 3 Interaction between various ASICs and P2X3Rs after their transfection into CHO cells. CHO cells were transfected with various ASICs and P2X3Rs in a 1:1 ratio or transfected only with rP2X3R or rASIC3, as indicated. Whole-cell patch-clamp recordings at a holding potential of −65 mV.a,bInteraction between hASIC3 and hP2X3Rs on their simultaneous activation. Interaction between rASIC1a (c) or rASIC2a (d) with rP2X3Rs on their simultaneous activation. The drug application and evaluation protocols were like those used in Fig.2a–g. Means ± S.E.M. of the indicated number of experiments. *P< 0.05; statistically significant difference between the current amplitudes before and after the shift in pH.§P < 0.05; statistically significant difference between the pH-induced inhibition of the current amplitudes at pH 4.0 and 3.5 (one-way ANOVA followed by the Bonferroni test in both cases).eCurrent responses were elicited in CHO-rASIC3/rP2X3R cells by α,β-meATP (10 µM) before, during and after the application of GMQ.fMeans ± S.E.M. percentage changes of the α,β-meATP-induced current responses were calculated with respect to the second current amplitude before GMQ application.gInhibition of current responses to α,β-meATP in CHO-rP2X3R cells.hMeans ± S.E.M. percentage inhibition in the indicated number of experiments as shown in (g).iNo change of the GMQ (1 mM)-induced current in the presence of α,β-meATP (10 µM) in CHO-rASIC3 cells.jMeans ± S.E.M. percentage change in the indicated number of experiments as shown in (i). *P< 0.05; statistically significant difference from the α,β-meATP-induced current amplitudes before GMQ application (one-way ANOVA followed by the Bonferroni or Mann–Whitney test, as appropriate). The scale labels for the vertical bars were 2 nA (a,g,i) and 1 nA (e). The scale labels for the horizontal bars were 50 s (a,e,g,i) Table 3 ). Alanine and double cysteine mutants were designed by QuickChange site-directed mutagenesis (Stratagene) according to the manufacturer’s protocol, and nucleotide sequences were verified by sequencing (IZKF, Leipzig). Culturing of CHO cells and transfection procedures CHO cells (Sigma-Aldrich) were cultured in Iscove’s medium (Biochrom) with 3.024 g/l NaHCO 3 , 10% fetal bovine serum (Biochrom) and 2 mM l -glutamin (Life Technologies) at 37 °C and 5% CO 2 in humidified air. For patch-clamp experiments cells were plated in plastic dishes. After a period of 6 h, 0.5 µg plasmid DNA (of ASIC and/or P2X3) was mixed with 10 µl Polyfect® transfection reagent (Qiagen) and 100 µl OptiMEM® (Invitrogen) for 10 min. Then, the lipid–DNA complexes were introduced to the cells in 500 µl Iscove’s medium. Approximately 16 h after transfection, Iscove’s medium was replaced by OptiMEM® to remove residual plasmid DNA. Culturing of rat dorsal root ganglion cells The present investigation was carried out in accordance with the national guidelines for the use of animals in biomedical research. One-day-old Wistar rats were decapitated and their thoracic and lumbar dorsal root ganglia were taken out and placed in Ca 2+ /Mg 2+ -free cold (4 °C) Hank’s balanced salt solution. The preparation of a cell suspension, its mechanical trituration and centrifugation to obtain a pellet was identical with that described earlier [57] . 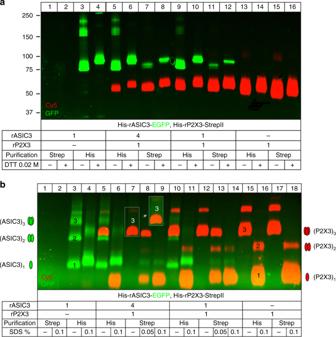Fig. 9 Plasma membrane expression and oligomeric assembly of rASIC3 and rP2X3R subunits in oocytes. For biochemical analysis,Xenopus (X.) laevisoocytes expressing the indicated proteins were surface labeled with the membrane-impermeant fluorescent Cy5 dye before protein purification. The indicated proteins were purified under non-denaturing conditions fromX. laevisoocytes by Ni2+-NTA chromatography or Strep-Tactin chromatography, as indicated, resolved by SDS-PAGE (a) or BN-PAGE (b), and visualized by Typhoon fluorescence scanning.aOverlay of the Cy5-labeled surface form (red) of the His-rASIC3-EGFP and His-rP2X3-StrepII protomers and the GFP fluorescence (green) of the His-rASIC3-EGFP protomer. The positions of molecular mass markers (in kDa) are shown on the left.bOverlay of GFP and Cy5 fluorescence of the homomeric His-rASIC3-EGFP (lanes 1–4) and homotrimeric His-rP2X3-StrepII (lanes 15–18) and the co-expressed His-rASIC3-EGFP and His-rP2X3-StrepII receptor subunits (lanes 5–14) in their native or partial SDS-denatured forms isolated by Ni2+-NTA (lanes 3–6, 10, 11, 15, 16) or Strep-Tactin (lanes 7–9, 12–14, 17, 18) chromatography as indicated. Co-expression of rASIC3 and rP2X3 (lanes 5–14) originates from the co-injection of the His-rASIC3-EGFP and His-rP2X3-StrepII subunit in cRNA ratios as indicated. The number of protomers included in the respective bands are exemplarily indicated. The inset shows the indicated section of the gel with enhanced GFP fluorescence to enable the visibility of the ASIC3 trimer. The schematics and labeling on the left or right margins indicate the numbers of rASIC3 or rP2X3 protomers incorporated in the respective trimeric (bold) or dimeric or monomeric protein band of the rASIC3 or rP2X3 receptor complexes, respectively 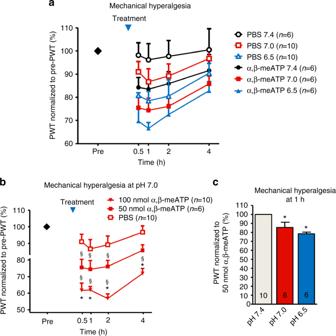Fig. 10 The effect of normal and pH-adjusted PBS solution and α,β-meATP on mechanical hyperalgesia in rats.aTime–response curves of the effect of intraplantar (i.pl.) phosphate-buffered saline (PBS) or α,β-meATP (50 nmol) dissolved in PBS injected into the right hind paw at a volume of 100 µl/paw on the baseline mechanical paw withdrawal threshold (PWT). Each point represents mean ± S.E.M. of the PWT in pressure as a percentage of baseline % applied to the hind paw before (pre) and after PBS/α,β-meATP administration, obtained from the indicated number of rats. α,β-meATP decreased PWT both pH and time dependently post injection (repeated measures ANOVA time × treatment effectF1,38= 1.760,P< 0.00001). The changes from baseline PWT were at pH 7.4, 16.5% (P= 0.0026,n= 6), at pH 7.0, 25.6% (P= 0.001,n= 6), at pH 6.5, 33.3% (P< 0.001,n= 6, one-way ANOVA followed by the Dunnett test) at 1 h. For the sake of clarity, statistical significance is not indicated in the figure.bDose-dependent effect of α,β-meATP on mechanical hyperalgesia at pH 7.0.§P < 0.05; statistically significant difference vs. baseline; *P< 0.05; statistically significant difference vs. PBS. Results were analyzed by repeated measures ANOVA, followed by Neuman–Keuls test,n= 6–10 animals per group.cThe effect of acidification on α,β-meATP-induced hyperalgesia. PWT values were normalized to the response obtained by 50 mM α,β-meATP at pH 7.4. *P< 0.05; statistically significant difference from the 100%. Results were analyzed by one-way ANOVA followed by Tukey test,n= 6 animals per group The obtained pellet was suspended in Dulbecco’s minimal essential medium supplemented with 30 ng/ml NGF, 10 ng/ml insulin, 5.5 µg/ml transferrin and 5 ng/ml selenium. DRG cells were plated at a density of 2 × 10 6 cells/ml on poly- l -lysin-coated culture dishes. Cultures were maintained for 2–4 days in humidified atmosphere at 37 °C in 5% CO 2 to reach a developmental stage without axonal sprouting. All culture media were from Invitrogen; additional drugs were from Sigma-Aldrich. Whole-cell patch-clamp recording and drug application Small DRG neurons (diameter <30 µm; 2–4 days of culturing) or transfected CHO cells (2 days after transfection with ASIC and/or P2X3 constructs) were chosen for whole-cell patch-clamp recordings at room temperature (20–22 °C) using an Axopach 200B patch-clamp amplifier (Molecular Devices). The pipette solution contained (in mM) CsCl 135, MgCl 2 2, HEPES 20, EGTA 11, CaCl 2 1, Mg-ATP 1.5 and Li-GTP 0.3; pH adjusted to 7.4 using CsOH. For the analysis of the effect of changes in intracellular Ca 2+ on the rASIC3 and rP2X3R current responses, the EGTA concentration was decreased to 1.1 mM or EGTA was replaced by 5 mM BAPTA in the pipette solution. When the reversal potential of rASIC3 was investigated, 10 mM NaCl was added to the intracellular solution and simultaneously the concentration of CsCl was decreased to 125 mM. The external physiological solution contained (in mM) NaCl 135, KCl 5, MgCl 2 2, CaCl 2 2, HEPES 10 and glucose 11; pH adjusted to 7.4 using NaOH. When the effect of changes in extracellular Ca 2+ concentration on rASIC3 and rP2X3 current amplitudes was analyzed, the CaCl 2 concentration was increased to 4 mM or Ca 2+ was omitted from the external physiological solution. The pipette resistances varied between 3 and 7 MΩ. Holding potential values given in this study were corrected for the liquid junction potential between the bath and pipette solution (−4.5 mV; calculated at 21 °C). All recordings were carried out at a holding potential of −65 mV, unless stated otherwise. Data were filtered at 2 kHz, digitized at 5 kHz and stored on a computer using a Digidata 1440 interface and the pClamp 10.2 software (Molecular Devices). Drugs were dissolved in the external physiological solution and locally superfused to single cells using the SF-77B Perfusion Fast-Step rapid solution exchange system (Warner Instruments). In all figures, the opening and/or closure of the application valves appear as small artifacts. The current responses to protons or α,β-meATP follow the opening of the valve with a certain delay depending on the dead space in the tubing of the application system and the position of the application pipette. Nonetheless, we indicated the period of drug application by drawing a horizontal line between the two artifacts. Immunofluorescence and confocal laser scanning microscopy DRG neurons were cultured for 48 h, as described previously, in the presence or absence of 30 ng/ml NGF [29] (Sigma-Aldrich). Cells were washed twice with Soerensen’s phosphate buffer (0.1 M, pH 7.4) and then fixated with 4% paraformaldehyde in the same buffer for 20 min at 4 °C. After washing cells twice with Tris-buffered saline (TBS, 0.05 M, pH 7.4), they were treated with blocking solution (TBS containing 5% fetal calf serum and 0.3% Triton X-100) and incubated overnight at 4 °C with the guinea pig anti-P2X3 antibody (1:400, Neuromics, cat. no. : GP 10108) and the rabbit anti-ASIC3 antibody (1:400, Alomone Labs, cat. no. : ASC-018). Cells were washed again three times with TBS before applying the Carbocyanine (Cy)2-conjugated donkey anti-guinea pig IgG (1:300) and the Cy3-conjugated donkey anti-rabbit IgG (1:800, both from Jackson ImmunoResearch) for 2 h at room temperature. Nuclei were stained with Hoechst 33342 (20 µg/ml in TBS, Invitrogen) for 10 min at room temperature and cells were washed again twice with TBS. Immunofluorescence was analyzed by a laser scanning microscope (LSM 510 Meta, Carl Zeiss) at excitation wavelengths of 488 nm (argon, green Cy2-fluorescence) and 543 nm (helium/neon 1, red Cy3-fluorescence), respectively. An ultraviolet laser (362 nm) was used to excite the blue-cyan Hoechst 33342 (auto) fluorescence. All antibodies were checked for target selectivity by using western blots and immunocytochemistry according to the product citations of the respective companies. Co-immunoprecipitation and western blot Primary rat DRG cultures were exposed to a buffer solution containing (in mM) 152 NaCl, 5 KCl, 1 MgCl 2 , 2 CaCl 2 , 10 glucose and 10 HEPES, pH adjusted to 7.4 or 6.8 with NaOH, for 3 min at room temperature, before cell lysis. For P2X3R silencing, cultures were treated either with scramble RNA or with siP2X3 RNA (Dharmacon) and used 72 h later. Where indicated, cells were thereafter treated with the crosslinker 3,3′-dithiobis sulfosuccinimidyl propionate (2 mM; DTSSP, spacer arm length: 12 Å; Thermo Fisher Scientific) for 30 min at 4 ° C and then lysed in a buffer containing 10 mM Tris, pH 7.5, 150 mM NaCl, 2 mM EDTA, 1% Triton X-100, 100 mM NaF, 20 mM sodium orthovanadate, plus a protease inhibitor mixture (Roche). Cell extracts were immunopurified with a rabbit anti-P2X3 antibody (Santa Cruz Biotechnology, cat. no. : sc-25694) and immunoblotted with rabbit anti-ASIC1, rabbit anti-ASIC2, rabbit anti-ASIC3, or rabbit anti-P2X3 antibodies (Alomone Labs, cat. nos. ASC-014, ASC-012, ASC-018 and APR-016, respectively). Gel loading was measured with mouse anti-β-Actin antibodies (Sigma-Aldrich, cat. no. : A3854). Immunoblot signals were visualized with a mouse anti-rabbit IgG light chain-specific antibody (Jackson ImmunoResearch, cat. no. : 211-002-171) and an enhanced chemiluminescence light system (GE Healthcare). For membrane protein biotinylation, CHO cells were co-transfected either with the ASIC3 plus EGFP-encoding plasmids or with P2X3 plus ASIC3-encoding plasmids (ratio 1:1) with Lipofectamine (Thermo Fisher Scientific) and after 24 h treated with membrane-impermeable biotin. Expression of the rASIC3 and rP2X3 subunits in oocytes An oocyte expression plasmid harboring the cDNA for the His 6 -tagged rP2X3 subunit was available from previous studies [30] , [58] . A StrepII affinity tag-encoding sequence 5′ of the stop codon of the His-hP2X3 construct was introduced by QuikChange site-directed mutagenesis. The rASIC3-encoding sequence was PCR-amplified from the rASIC3-pEGFP-C3 plasmid described above and subcloned into a Gateway-modified version of the oocyte expression vector pNKS2. A His 8 affinity tag-encoding sequence 3′ of the start codon of the rASIC3 construct was introduced by QuikChange site-directed mutagenesis. An EGFP-encoding sequence was PCR-amplified from the pIRES2-EGFP vector (Clontech) and introduced 5′ of the stop codon of the His-rASIC3 construct by domain-swapping using the Mega-primer method [59] . Primers are listed in Suppl. Table 3 . All cDNA constructs were verified by nucleotide sequencing (MWG Germany). Capped cRNAs were synthesized and injected in aliquots of 50 nl (1 ng/nl or 0.1 ng/nl for biochemical analysis or two-electrode voltage-clamp experiments, respectively) into collagenase-defolliculated X. laevis oocytes using a Nanoliter 2000 injector (World Precision Instruments). For co-expression of the rASIC3 and rP2X3R subunits, the His-rASIC3-EGFP and His-rP2X3-StrepII encoding cRNAs were co-injected at 1:1 or 4:1 ratios (w/w), respectively. Oocytes were cultured at 19 °C in sterile oocyte Ringer’s solution (in mM: NaCl 90, KCl 1, CaCl 2 1, MgCl 2 1, and HEPES 10, pH 7.4) supplemented with 50 µg/ml of gentamycin. Two-electrode voltage-clamp electrophysiology At 1 to 2 days after cRNA injection, oocytes were incubated at room temperature (21–24 °C) in Mg-Ori solution (in mM): NaCl 90, KCl 1, MgCl 2 2 and HEPES 10 (pH 7.4) or MES 10 (pH 6.5). Current responses were evoked by α,β-meATP and recorded by conventional two-electrode voltage-clamp (TEVC) with a Turbo TEC-05 amplifier (npi Electronics) at a holding potential of −60 mV [58] . For analysis of the interaction of the rP2X3R and the rASIC3, oocytes expressing the rP2X3R (control) or co-expressing the rP2X3R and the rASIC3 were superfused with 3 or 10 µM α,β-meATP nine times for 5 s in 3 min intervals. After the third α,β-meATP application (first application not shown) the pH value of the Mg-ORi solution was shifted from 7.4 to 6.5 for three intervals and three α,β-meATP applications, which was followed by three subsequent applications of the original α,β-meATP concentration at pH 7.4. Biochemical analysis of subunit oligomerisation in ocytes The cRNA-injected oocytes were metabolically labeled by overnight incubation with l -[ 35 S]methionine (Perkin Elmer Life Sciences) and, after an additional 24 h chase period, just before protein extraction, surface labeled with the membrane-impermeant fluorescent dye Cy5-NHS ester (50 µg/ml, GE Healthcare Biosciences) in PBS at pH 8.5 (in mM: 20 sodium phosphate, 110 NaCl, 1 MgCl 2 ), and then incubated for 30 min at ambient temperature (21–24 °C). Affinity-tagged proteins were purified by non-denaturing Ni 2+ -NTA chromatography (Qiagen) or Strep-Tactin chromatography (IBA Germany) from n-dodecyl-beta-D-maltoside (DDM, 0.2%, w/v) extracts of the oocytes as indicated. An elution buffer consisting of 0.5% (w/v) digitonin in 250 mM imidazole/HCl (pH 7.6) or 0.5% (w/v) digitonin in 0.1 M sodium phosphate buffer, pH 8.0 supplemented with 10 mM biotin, respectively, was used to release the proteins in the non-denatured state from the Ni 2+ -NTA sepharose or the Strep-Tactin sepharose. The proteins were analyzed by BN-PAGE or SDS-PAGE in the non-denatured or SDS-denatured state, respectively [26] . Where indicated, samples were treated before BN-PAGE (4–14 % acrylamide) for 1 h at 37 °C with 0.05 or 0.1% (w/v) SDS to induce partial dissociation of the rP2X3 and rASIC3 receptor complexes. The Cy5-labeled plasma membrane-bound proteins and the EGFP-tagged rASIC3 subunits were visualized by a Typhoon 9410 fluorescence scanner (GE Healthcare). Images of PAGE-gels were prepared with the ImageQuant software for contrast adjustments. The image sections were cropped and positioned using Adobe Photoshop CS5. Microsoft PowerPoint 2013 was used for labeling. Measurement of mechanical hyperalgesia Male Wistar rats (250–300 g; Toxicoop) were used in nociceptive behavior experiments. All procedures on animals were approved and reviewed by the local Animal Care Committee of the Institute of Experimental Medicine (Budapest, Hungary). Animals were randomly assigned to experimental groups and subsequent drug treatment and behavioral analyses were performed blindly. α,β-meATP was prepared in normal (pH 7.4) or pH-adjusted (pH 7.0 and 6.5) PBS. Rats were anesthetised with isoflurane and injected i. pl. into the central sole region of the right hind paw with 100 µl PBS or α,β-meATP using a 25-gauge needle. The animals were then tested behaviorally for their responses to mechanical stimulations. Mechanical sensitivity of rats was assessed by measuring PWT using a calibrated electronic von Frey apparatus (Dynamic plantar anesthesiometer, Ugo Basile Instruments) on each animal before and after i.pl. treatment. Rats were placed on a metal mesh grid under a plastic observation chamber and habituated for 10 min. Ten measurements at approximately 20 s intervals were taken from each hind paw and then paw withdrawal responses to each set of 10 stimuli was averaged to determine PWT, expressed in grams. After the measurement of the baseline PWT, rats were anesthetized and normal or pH-adjusted PBS or α,β-meATP was injected subcutaneously into the plantar surface of right hind paw. PWT was measured at 0.5, 1, 2 and 4 h after the injection. The mechanical hyperalgesia in each experimental animal was presented as a percentage of baseline PWT. Data analysis Concentration–reponse curves were fitted with the Origin 8.0 (OriginLab) software using the three-parametric Hill equation: 
    I = I_max· [A]^nH/(EC_50^nH + [A]^nH),
 (1) where I represents the peak current elicited by a certain concentration of H + or α,β-meATP [A] , I max is the peak current evoked by the maximal effective concentration of H + or α,β-meATP, EC 50 is the half maximal effective concentration of H + or α,β-meATP and n H is the Hill coefficient. In contrast to the calculated I max , we designed the measured maxima of the curves as I mean (see concentration–response curves in each figure). Current–voltage plots were constructed by plotting current responses against the holding potentials and using a linear fit with the equation: 
    y = m · x + n.
 (2) The reversal potential ( x ) was calculated at y = 0 . To analyze the interaction between two ion channels after co-transfection of P2X3 with ASIC3, ASIC1a or ASIC2a, current responses elicited by α,β-meATP were compared before, after and during the pH shift. For this purpose, the mean value calculated from the second and third current responses during the pH shift were normalized to the current amplitude immediately before the shift at pH 7.4, which was set at 100%. The figures show mean ± S.E.M. of multiple ( n ) experiments carried out on separate cells. A sample size of six or more was chosen to ensure adequate power to detect a pre-specified effect size. Statistically significant differences between I max , I mean , EC 50 , and n H values derived from concentration–response curves were analyzed by one-way analysis of variance (ANOVA) followed by the Holm–Sidak post hoc test. The effect of the potentiation of the current through one ion channel (e.g., P2X3R) by co-activation of the other ion channel (e.g., ASIC3) was evaluated by one-way ANOVA followed by the Bonferroni post hoc test. When two values were compared with each other, Student’s t -test (normal distribution) and the Mann–Whitney test (non-normal distribution) was used, as appropriate. A probability level of P < 0.05 or less was considered to reflect a statistically significant difference. In behavioral studies, all data were expressed as means ± S.E.M. of n observations, where n means number of animals per group. Behavioral data were statistically tested using a repeated measures ANOVA to determine the overall effect of treatment and time; for post hoc analysis, Newman–Keuls multiple comparison test was performed to determine significant differences among groups (STATISTICA software). A value of P < 0.05 was considered to be statistically significant. Data availability Data supporting the findings of this manuscript are available from the corresponding author upon reasonable request.